Polyploid cells rewire DNA damage response networks to overcome replication stress-induced barriers for tumour progression Mutations in genes involved in DNA replication, such as flap endonuclease 1 ( FEN1 ), can cause single-stranded DNA breaks (SSBs) and subsequent collapse of DNA replication forks leading to DNA replication stresses. Persistent replication stresses normally induce p53-mediated senescence or apoptosis to prevent tumour progression. It is unclear how some mutant cells can overcome persistent replication stresses and bypass the p53-mediated pathways to develop malignancy. Here we show that polyploidy, which is often observed in human cancers, leads to overexpression of BRCA1 , p19arf and other DNA repair genes in FEN1 mutant cells. This overexpression triggers SSB repair and non-homologous end-joining pathways to increase DNA repair activity, but at the cost of frequent chromosomal translocations. Meanwhile, DNA methylation silences p53 target genes to bypass the p53-mediated senescence and apoptosis. These molecular changes rewire DNA damage response and repair gene networks in polyploid tumour cells, enabling them to escape replication stress-induced senescence barriers. DNA single-strand breaks (SSBs) frequently occur during DNA replication and repair [1] . The most well-known example occurs during replication of the lagging DNA strand, a process in which millions of short DNA fragments (Okazaki fragments) are synthesised. Okazaki fragments are processed by the combined action of DNA polymerase δ, flap endonuclease 1 (FEN1) and DNA ligase 1, which seal the nicks between each fragment to produce the intact lagging DNA strand [2] , [3] , [4] . Mutations in any one of these genes, including FEN1 , can impair Okazaki fragment maturation, leading to persistent DNA SSBs in the genome [1] , [5] , [6] . In addition, SSBs or gaps are transiently produced by nuclease cleavage during DNA repair, including mismatch repair, nucleotide excision repair and base excision repair [1] , [5] , [6] . Furthermore, SSBs may also arise directly after exposure to DNA damaging agents such as ionising radiation [1] . Mammalian cells have evolved DNA SSB repair pathways and are relatively tolerant to SSBs. Critically, however, unrepaired DNA SSBs can collapse DNA replication forks, leading to replication stresses and one-ended DNA double-strand breaks (DSBs), which are the most challenging lesions for cells to repair [1] , [7] , [8] . Cells have evolved multiple DNA damage response and repair pathways to deal with collapsed replication forks and DSBs to prevent transmission of DNA damage and genome instabilities to daughter cells. In response to collapsed replication forks, cells activate DNA checkpoints and arrest cell cycle progression to allow the repair of the stalled forks. Accurate repair of the one-ended DSBs and restart of the collapsed replication fork require the homologous recombination (HR) repair machinery and a homologous DNA sequence as the repair template [7] , [8] . In rare cases, a one-ended DSB may be misaligned with another DSB and misjoined by the non-homologous end-joining (NHEJ) machinery [7] . This misjoining results in chromosomal translocations, which are among the most common cytogenetic aberrations in cancer cells [9] . Because faithful duplication and transmission of the chromosomes into daughter cells is critical for the survival of organisms, it is thought that NHEJ complexes are inhibited at one-ended DNA DSBs [7] . In the case of continued DNA-replication stress and persistent formation of DSBs, p53-mediated cellular senescence or apoptosis is induced to prevent proliferation of damaged cells [10] , [11] , [12] . It is unclear how tumour cells breach this replication-stress-mediated barrier and progress into malignant cancers. To address this question, we used a previously established mutant mouse model carrying a point mutation (F343A/F344A, FFAA) in the FEN1 gene that encodes an endonuclease critical for the Okazaki fragment maturation [6] , [13] . Mutant FFAA mouse cells display defects in the Okazaki fragment maturation and consequently high levels of unligated DNA SSBs and DSBs [6] . These cells also have high potential to become tetraploid and aneuploid [6] . Here we show that the near-polyploid aneuploid cancer cells can induce epigenetic changes that lead to the overexpression of BRCA1 , p19arf and other DNA repair genes, but downregulate p53 target genes in the senescence and apoptosis pathways. As a consequence, the DNA damage response and repair networks are rewired in the near-polyploid aneuploid cancer cells, leading to reduction of DNA replication stresses and escaping of senescence and apoptosis. Polyploid tumour cells overcome ATR-mediated senescence We previously showed that heterozygous mutant mice harbouring the FFAA mutation in FEN1 , which causes defects in the Okazaki fragment maturation were prone to the development of malignant cancers [6] , [13] . To determine how WT/FFAA cells develop malignancy, we examined their response to DNA replication stresses and sought to identify the underlying molecular events. Previously, we showed that primary WT/FFAA mouse embryonic fibroblasts (MEFs) grown in normal culture conditions have the capacity to form large numbers of foci [6] . Cells from these foci were thought to be tumour-initiating cells [14] , [15] . To characterise these tumour-initiating cells, we conducted serial expansion of these cells ( Fig. 1a ). We found that 23% of the foci could expand unlimitedly with the remaining 77%, displaying only limited clonal expansion capability. The unlimitedly expanding cells displayed a fast and unrestricted proliferation, compared with the normal diploid MEF cells, which showed a gradually deceased proliferation ( Fig. 1b ). Consistently, they had significantly higher proportions of S- and G2-phase cells than those of primary diploid WT/FFAA MEF cells ( Supplementary Fig S1 ), and formed subcutaneous cancers in the immunodeficient NOD/SCID mice. In contrast, cells capable of only limited expansion showed little growth at 10–15 days ( Fig. 1b ). Previously, the FFAA FEN1 mutation was shown to induce tetraploidy [6] , which presumably causes more DNA replication stresses due to the high DNA content of the tetraploid cells. To determine if tetraploidy was associated with the expansion phenotypes of WT/FFAA tumour cells, we counted the chromosome number of these two types of tumour cells. Surprisingly, all the unlimitedly expanding clones had near-polyploid aneuploidy (hereafter referred to as aneuploidy; Fig. 1c and Supplementary Fig. S2 ). In contrast, cells of three limitedly expanding clones were diploid or near-diploid ( Fig. 1c ). 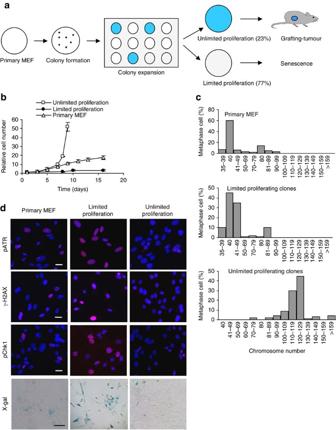Figure 1: Selection of near-polyploid aneuploid cells clonal expansion under oncogenesis-induced DNA replication stresses. (a) Cartoon of expansion method for spontaneously formed colonies of WT/FFAA MEFs. Cells from a single colony were cultured in a 48-well plate. Once the cell culture reached 90% confluence, the cells were further expanded in 24-, 12- and 6-well plates, or 10-cm dishes. Colonies that expanded for at least 10 passages without a decrease in proliferation rate were considered unlimited expansion clones, and were confirmed to form cancers in NOD/SCID mice. (b) Growth rates of diploid MEF cells, limited and unlimited expansion colonies. Values are means±s.d. of five independent clones. (c) Chromosome numbers of primary WT/FFAA MEF cells (P0) and representative clones with limited or unlimited expansion at the 6-well plate stage were counted using metaphase spread. More than 100 mitotic cells were analysed for each spread. (d) Upper panels: primary WT/FFAA MEF cells and tumour cells from limitedly and unlimitedly proliferating clones stained for the phosphorylated forms of ATR, H2AX and Chk1 (red). Nuclei were stained with DAPI (blue). Scale bar equals 25 μm. Lower panels: detection of senescent cells by X-gal staining (blue). Scale bar equals 100 μm. Figure 1: Selection of near-polyploid aneuploid cells clonal expansion under oncogenesis-induced DNA replication stresses. ( a ) Cartoon of expansion method for spontaneously formed colonies of WT/FFAA MEFs. Cells from a single colony were cultured in a 48-well plate. Once the cell culture reached 90% confluence, the cells were further expanded in 24-, 12- and 6-well plates, or 10-cm dishes. Colonies that expanded for at least 10 passages without a decrease in proliferation rate were considered unlimited expansion clones, and were confirmed to form cancers in NOD/SCID mice. ( b ) Growth rates of diploid MEF cells, limited and unlimited expansion colonies. Values are means±s.d. of five independent clones. ( c ) Chromosome numbers of primary WT/FFAA MEF cells (P0) and representative clones with limited or unlimited expansion at the 6-well plate stage were counted using metaphase spread. More than 100 mitotic cells were analysed for each spread. ( d ) Upper panels: primary WT/FFAA MEF cells and tumour cells from limitedly and unlimitedly proliferating clones stained for the phosphorylated forms of ATR, H2AX and Chk1 (red). Nuclei were stained with DAPI (blue). Scale bar equals 25 μm. Lower panels: detection of senescent cells by X-gal staining (blue). Scale bar equals 100 μm. Full size image To determine the activation of DNA damage response pathways and cellular senescence in primary WT/FFAA MEFs, and the limitedly or unlimitedly expanding tumour cells, we immunofluorescently stained the cells for the phosphorylated (activated) forms of ATM, ATR, H2AX, Chk1 and Chk2. Previously, we showed that the FFAA mutation caused DNA replication defects that activated ATR and Chk1 [6] ( Fig. 1d ). A number of the primary WT/FFAA cells were positive for X-gal staining, which was the indicator for cellular senescence ( Fig. 1d ). Near-diploid tumour cells of limited expansion were positive for phosphorylated ATR-, γH2AX- and Chk1 ( Fig. 1d ), but unexpectedly, were negative for phospho-ATM and -Chk2. X-gal staining also showed that tumour cells in the limitedly expanding clones were predominantly senescent ( Fig. 1d ). In contrast, very few of the aneuploid tumour cells of unlimited expansion showed activation of these DNA damage response proteins, and they did not undergo cellular senescence ( Fig. 1d ). Polyploid tumour cells alter DNA damage response pathways To search for the molecular mechanisms driving how the aneuploid cancer cells overcome DNA replication stresses and abrogate DNA damage responses and cellular senescence, we used mRNA microarray analysis to compare genome-wide gene expression profiling of primary WT/FFAA MEF cells (control) with that of the tumour cells having limited or unlimited proliferation potential. A total of 79 genes were upregulated and 121 downregulated in the senescent tumour cells, compared with the normal control. Ingenuity pathway analysis indicated cancer as the most relevant disease, confirming that these cells were indeed tumour-related. Furthermore, CXCL2-centered cytokine signalling was the only significantly upregulated gene network in the limitedly expanding tumour cells ( Fig. 2 ). The most upregulated gene CXCL2 (15-fold) is a ligand of CXCR2, which has a key role in reinforcement of ATM/ATR-mediated oncogenesis-induced senescence [16] . In contrast to the senescent tumour cells, expression of CXCL2 and other related chemokine-signalling genes was significantly downregulated in the expanding aneuploid cancer cells ( Fig. 2 ). This suggested that the aneuploid cancer cells may downregulate CXCL2-mediated signalling to attenuate ATR-mediated oncogenesis-induced senescence. 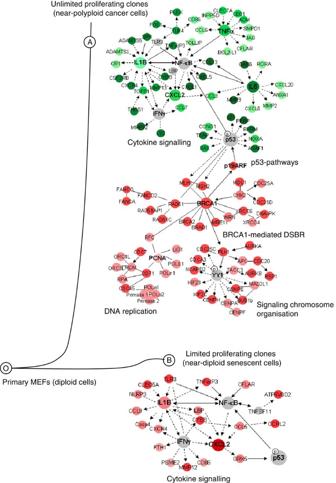Figure 2: Gene expression analysis of near-polyploid aneuploid cancer cells. Microarray gene expression profiling analysis of primary WT/FFAA diploid control cells (O), or tumour cells with limited expansion (B) or unlimited expansion (A). Microarray hybridisation data analysed with Ingenuity Pathway analysis identified significantly relevant disorders and upregulated or downregulated gene networks or pathways, compared with the diploid control. Red circles, upregulated genes; green circles, downregulated genes; solid lines, physical interaction; arrows with dashed lines, induction of gene expression; arrows with solid lines, activation. The degree of the change in expression is qualitatively reflected by the darkness of the color. DSBR: DSB repair. Figure 2: Gene expression analysis of near-polyploid aneuploid cancer cells. Microarray gene expression profiling analysis of primary WT/FFAA diploid control cells (O), or tumour cells with limited expansion (B) or unlimited expansion (A). Microarray hybridisation data analysed with Ingenuity Pathway analysis identified significantly relevant disorders and upregulated or downregulated gene networks or pathways, compared with the diploid control. Red circles, upregulated genes; green circles, downregulated genes; solid lines, physical interaction; arrows with dashed lines, induction of gene expression; arrows with solid lines, activation. The degree of the change in expression is qualitatively reflected by the darkness of the color. DSBR: DSB repair. Full size image Approximately 1,400 genes were significantly upregulated in the aneuploid cancer cells compared with the control cells. The highly upregulated gene networks were DNA replication, chromosome organisation and DNA repair genes for the HR, NHEJ, BER and MMR pathways ( Fig. 2 and Supplementary Table S1 ). In addition to DNA repair genes, the cell-cycle checkpoint genes BRCA1 and p19arf were significantly upregulated. This increased expression was confirmed by quantitative real-time PCR, because the number of mRNAs of BRCA1 and p19arf per gene copy in the aneuploid cancer cells was significantly higher than in the control diploid cells ( Supplementary Fig. S3 ). BRCA1 is central to the upregulated DNA-repair networks interacting with other DNA-repair proteins such as Rad51 and the Fanconi Anemia proteins, and it is thought to be important for various DSB-repair pathways ( Fig. 2 ) [17] , [18] , [19] , [20] . BRCA1 also interacts with the tumour suppressor gene p19arf to stabilise p53 and induce the expression of p21, resulting in cellular senescence [21] , [22] , [23] . Interestingly, we noticed that p21 and other p53 target genes were significantly downregulated in the aneuploid cancer cells ( Fig. 2 and Supplementary Table S2 ), suggesting that the activation of BRCA1 and p19arf, and expression of p21 were uncoupled in the aneuploid cancer cells. Therefore, the transcriptome profiling analysis suggested the BRCA1- and p19arf-mediated DNA damage response and repair networks, which could facilitate DNA repair but suppress senescence or apoptosis. Overexpression of BRCA1 and p19arf enhances DNA SSB repair We next investigated if overexpression of BRCA1 and p19arf was induced by polyploidisation. We used fluorescence-activated cell sorting (FACS) to separate the tetraploid cell population from the diploid one, which had similar cell-cycle profiling to each other ( Supplementary Fig. S4a and 4b ). Because the primary tetraploid cells are genetically and epigenetically unstable [24] , it seemed possible that not all tetraploid cells overexpressed BRCA1 and p19arf. A microfluidic device was used to capture single cells from the FACS-sorted diploid or tetraploid cell populations, most of which were at the G1/G0 phase ( Supplementary Fig. S4 ). Expression profiling of BRCA1 and p19arf was determined at the single-cell level. The diploid WT/FFAA cells, which were previously shown to have increased numbers of DNA SSBs and DSBs [6] , expressed low levels of BRCA1 or p19arf in a relatively uniform manner ( Supplementary Fig. S5 ), suggesting that DNA damage due to the FFAA FEN1 mutation is not responsible for the overexpression of BRCA1 and p19arf. In contrast, the tetraploid cells overexpressed BRCA1 or p19arf in a heterogeneous fashion ( Supplementary Fig. S5 ). The heterogeneous overexpression of BRCA1 and p19arf in primary tetraploid cells was confirmed by in situ ViewRNA analysis ( Supplementary Fig. S6 ). Interestingly, all the aneuploid cancer cells uniformly overexpressed both BRCA1 and p19arf ( Supplementary Fig. S6 ). It seems possible, therefore, that tetraploidy could result in the heterogeneous induction of BRCA1 and/or p19arf, and that the cells that overexpress both BRCA1 and p19arf are selected for during clonal expansion. Next, we investigated the role of overexpression of BRCA1 and p19arf in coping with DNA replication stresses. One possible mechanism is that it promotes the repair of DNA SSBs that arise due to FEN1 FFAA mutation as well as oncogenesis-induced hyper-DNA replication. To evaluate if the aneuploid cancer cells that overexpressed both BRCA1 and p19arf had a greater capacity for repairing DNA SSBs than did the diploid MEFs, nuclear extracts (NEs) were prepared from both cell types and assayed the DNA SSB repair efficiencies, using two gapped DNA substrates representing DNA SSB intermediate structures that occur during Okazaki fragment maturation or long-patch BER ( Fig. 3a,b ). NEs from the aneuploid cancer cells generated considerably more fully repaired products than did NEs from the primary diploid MEFs ( Fig. 3a,b ). However, adding BRCA1 or p19arf antibodies to NEs from the aneuploid cancer cells reduced the in vitro SSB repair efficiency by more than 90% ( Fig. 3c,d ). It indicated that that BRCA1 and p19arf have important roles in stimulating DNA SSB repair in these cells. To further elucidate how BRCA1 and p19arf contribute to SSB repair, the effect of BRCA1 and p19arf on gap filling mediated by Polδ and Polβ, which are essential steps during DNA SSB repair [1] , [5] , was analysed. We found that recombinant human BRCA1 could slightly (approximately two-fold) stimulate human Polδ and Polβ to incorporate 32 P-dCTP into a gapped DNA duplex, whereas recombinant human p14arf protein, the mouse p19arf homologue, greatly enhanced the gap-filling activity ( Supplementary Fig S7a, b ). In addition, both BRCA1 and p14arf enhanced FEN1-mediated flap cleavage ( Supplementary Fig. S8 ), which occurs during Okazaki fragment maturation, and can also occur during LB-BER, DNA SSB repair and NHEJ [4] , [5] , [25] , [26] , [27] . Small interfering RNA (siRNA) to knockdown BRCA1 or p19arf expression in the aneuploid cancer cells ( Supplementary Fig. S9a,b ) showed that the number of γH2AX-foci per nuclei was greatly increased in the aneuploid cancer cells treated with BRCA1 or p19arf siRNA ( Fig. 3e ). Knockdown of BRCA1 or p19arf also arrested the growth of the aneuploid cancer cells ( Supplementary Fig. S9c ). 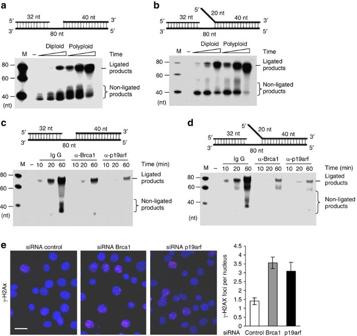Figure 3: BRCA1 and p19arf are crucial for DNA SSB repair and reduction of DNA DSBs. A gapped DNA substrate (a) or a gapped DNA flap substrate(b)(upper panels) was used to assay the NEs of primary diploid MEFs (P0) or the aneuploid cancer cells. A quantity 2 μg of each NE was incubated with the indicated DNA substrates (1 pmol). All reactions were carried under conditions described in methods for 10, 20 and 60 min, then analysed by 15% denaturing PAGE. (c,d) Reactions to assess SSB repair using NEs from the aneuploid cancer cells were carried out as described for (a) and (b), except that mouse IgG (400 ng) against Brca1 or p19arf was added to block their function. Non-specific mouse IgG (400 ng) was added for the controls (e) Aneuploid cancer cells with siRNA-mediated knockdown of BRCA1 or p19arf were stained for γ-H2AX (red) to evaluate DNA damage. Nuclei were stained with DAPI (blue). Left panel: γ-H2AX staining. Right panel: quantification of γ-H2AX foci per nuclei. The total number of γ-H2AX foci was normalised with the total number of nuclei. Values are mean±s.d.,n=3 independent assays. Scale bar equals 25 μm. Figure 3: BRCA1 and p19arf are crucial for DNA SSB repair and reduction of DNA DSBs. A gapped DNA substrate ( a ) or a gapped DNA flap substrate (b) (upper panels) was used to assay the NEs of primary diploid MEFs (P0) or the aneuploid cancer cells. A quantity 2 μg of each NE was incubated with the indicated DNA substrates (1 pmol). All reactions were carried under conditions described in methods for 10, 20 and 60 min, then analysed by 15% denaturing PAGE. ( c , d ) Reactions to assess SSB repair using NEs from the aneuploid cancer cells were carried out as described for ( a ) and ( b ), except that mouse IgG (400 ng) against Brca1 or p19arf was added to block their function. Non-specific mouse IgG (400 ng) was added for the controls ( e ) Aneuploid cancer cells with siRNA-mediated knockdown of BRCA1 or p19arf were stained for γ-H2AX (red) to evaluate DNA damage. Nuclei were stained with DAPI (blue). Left panel: γ-H2AX staining. Right panel: quantification of γ-H2AX foci per nuclei. The total number of γ-H2AX foci was normalised with the total number of nuclei. Values are mean±s.d., n =3 independent assays. Scale bar equals 25 μm. Full size image The NHEJ pathway is stimulated in polyploid cancer cells We noticed that the levels of some DNA repair genes that are involved in the NHEJ pathway, including DNA-PK, WRN and XRCC4 [7] , were increased in the near-polyploid aneuploid cancer cells ( Fig. 2 ). To determine if the aneuploid cancer cells had an enhanced NHEJ activity, we assayed the NHEJ activity of NEs from normal MEFs or aneuploid cancer cells using a synthetic oligo-based substrate with non-compatible 3′ ends [28] . The NHEJ activity of the NEs from the aneuploid cancer cell was increased by more than 20-fold compared to the NEs from primary MEFs, which had little NHEJ activity on these non-compatible DNA ends ( Fig. 4a ). Although the increase in NHEJ activity should allow the tumour cells to repair DSBs and suppress DSB-induced cellular senescence or apoptosis, at the same time, it could also lead to misjoining the one-ended DNA DSBs with other DSBs. In support of this hypothesis, all of the WT/FFAA aneuploid cancer cells had chromosome translocations, but none in the diploid WT/FFAA cells ( Fig. 4b ). Adding BRCA1 or p19arf antibodies to the NEs also inhibited the NHEJ activity on non-compatible DNA ends, albeit at a moderate level ( Fig. 4c ). 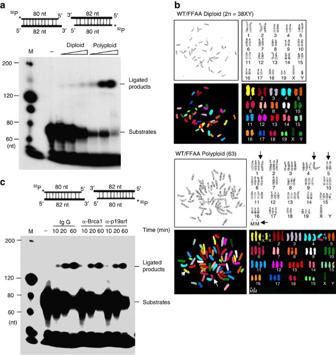Figure 4: Near-polyploid aneuploid cancer cells promote the NHEJ activity and cause chromosome translocations. (a) NHEJ activity of NEs from the diploid normal and aneuploid cancer cells. A32P-labeled DNA duplex with a two nucleotide 3′-end overhang was prepared (upper panel) and incubated with the indicated NEs (4 μg each) under conditions described in methods for 10, 20 and 60 min, and analysed by 6% denaturing PAGE. (b) GTG (upper panels) and SKY (lower panels) karyotypes of chromosomes in primary WT/FFAA MEFs or aneuploid cancer cells (clone C21). Structural chromosome aberrations, including two dicentric chromosomes composed of material from chromosome 1 and chromosome X (Dic(1H1;XA1)), and material from chromosome 4 and chromosome 18 (Dic(4C7, 18E4)), two inversions of chromosome 5 (In(5B-F)), and two additional micro-chromosomes, are indicated by arrows. (c) Reactions to assess NHEJ activities using NEs from the aneuploid cancer cells were carried out as described in (a), except mouse IgG againstBRCA1orp19arfwas added to block their function. Non-specific mouse IgG was used for control reactions. Figure 4: Near-polyploid aneuploid cancer cells promote the NHEJ activity and cause chromosome translocations. ( a ) NHEJ activity of NEs from the diploid normal and aneuploid cancer cells. A 32 P-labeled DNA duplex with a two nucleotide 3′-end overhang was prepared (upper panel) and incubated with the indicated NEs (4 μg each) under conditions described in methods for 10, 20 and 60 min, and analysed by 6% denaturing PAGE. ( b ) GTG (upper panels) and SKY (lower panels) karyotypes of chromosomes in primary WT/FFAA MEFs or aneuploid cancer cells (clone C21). Structural chromosome aberrations, including two dicentric chromosomes composed of material from chromosome 1 and chromosome X (Dic(1H1;XA1)), and material from chromosome 4 and chromosome 18 (Dic(4C7, 18E4)), two inversions of chromosome 5 (In(5B-F)), and two additional micro-chromosomes, are indicated by arrows. ( c ) Reactions to assess NHEJ activities using NEs from the aneuploid cancer cells were carried out as described in ( a ), except mouse IgG against BRCA1 or p19arf was added to block their function. Non-specific mouse IgG was used for control reactions. Full size image Epigenetic silencing of p21 abrogates cellular senescence BRCA1 and p19arf, on the other hand, may also activate p53, which induces the expression of downstream effectors such as p21, to limit the proliferation of aneuploid cancer cells [21] , [22] , [23] , [29] . Activation of p53 in WT/FFAA aneuploid cancer cells was confirmed by western blot analysis showing that the levels of nuclear p53 and phosphorylated-p53 were considerably elevated ( Fig. 5a ). This result led us to question how the cancer cells employed increased levels of BRCA1 and p19arf to reduce DNA replication stresses, yet avoided BRCA1-, p19arf- and p53-mediated cellular senescence and apoptosis. Our microarray data indicated that p21 was downregulated ( Fig. 2 ). Because p21 is a key effector gene downstream of the BRCA1–p19arf–p53 pathway [30] , [31] , [32] , this event might be crucial for enabling the tumour cells to escape BRCA1–p19arf–p53-mediated cellular senescence. Western blot analysis confirmed that the activation of p53 and expression of p21 were uncoupled in the aneuploid cancer cells ( Fig. 5a ). We searched for DNA mutations in the coding region and boundary regions between the exons and introns of p53 . However, we did not detect any mutations or deletions of the p53 gene in the aneuploid cancer cell lines or in lung tumours, suggesting that other mechanisms, such as epigenetic changes, were allowing the cells to bypass the p53-mediated barriers [33] . Supporting this hypothesis, we found that DNA methylation occurred in CpG islands in the promoter regions of the p53 target genes p21, PERP and RPRM ( Fig. 5b and Supplementary Fig. S10 ). To further test our hypothesis that DNA methylation contributed to the downregulation of p21 , we treated the aneuploid cancer cells and diploid normal cells with the DNA methylation inhibitor 5-aza-2′-deoxycytidine (5-AzadC; 500 ng ml −1 ), and this treatment restored p21 expression in the aneuploid cancer cells ( Fig. 5c,d ). Consistently, 5′ AzadC suppressed the proliferation of aneuploid cancer cells, but not of the primary MEFs ( Fig. 5e ). To further test if DNA methylation silencing of p21 was indeed a key factor in the ability of the aneuploid cancer cells to evade growth arrest, we pre-treated the cells with siRNA specific to p21 and then cultured them in the absence or presence of 5′ AzadC. We found that 5′ AzadC significantly inhibited the growth of the aneuploid cells treated with a control siRNA, but this effect was largely reversed in cells treated with p21 siRNA and 5′ AzadC ( Fig. 5f ). Furthermore, we showed that the expression of exogenous p21 in the aneuploid cancer cells resulted in an obvious growth inhibition ( Fig. 5g ). 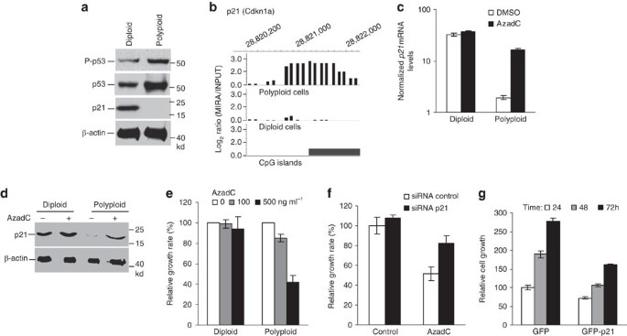Figure 5: DNA methylation silencing of p21 uncouples p53 activation and p21 expression. (a) Western blot analyses of levels of the nuclear form of p53, phosphorylated p53 (P-p53), and p21 in the normal diploid and aneuploid cancer cells. (b) DNA methylation status in the promoter regions ofp21(Cdkn1a) in aneuploid cancer cells and normal diploid cells. DNA methylation status is indicated by the Log2value of the hybridisation signal from the enriched methylated genomic DNA (MIRA) normalised with that from the input genomic DNA (INPUT). Black bars, hybridisation signals; grey bar, location of CpG islands. The DNA methylation profiling data accession number: GSE18815. (c,d) Near-polyploid aneuploid cancer or diploid normal cells (n=3 for each type) were treated with 5′ AzadC (500 ng ml−1) for 48 h. The mRNA (c) and protein levels (d) ofp21in the 5′ AzadC-treated or untreated cells were analysed by quantitative PCR and western blot analysis, respectively. (e)Aneuploid cancer or diploid normal cells were treated with 5′ AzadC (0, 100, or 500 ng ml−1; 48 h). Live cells were counted, and the relative growth rate calculated by dividing the number of cells by the number of the untreated cells (mock). Values are means±s.d. of three independent assays. (f) Aneuploid cancer cells were pretreated with control or p21 siRNA then cultured in the absence or presence of 500 ng ml−15′ AzadC for 48 h. The cell number was counted and the relative growth rate was calculated by dividing the number of cells under varying treatments by the number of cells treated with control siRNA oligos only. (g) Near-polyploid aneuploid cancer cells expressing GFP or GFP-p21 were seeded in 96-well plates (4,000 each well). Cell growth was monitored by CellTiter 96 Aqueous One Solution Cell Proliferation Assay kit every 24 h for 72 h. The relative cell number was calculated by comparison of the absorbance value at 570 nm (A570) of each well. The relative cell number of the wells with the cells expressing GFP only at 24 h was set as 100. Values are mean±s.d. ofn=5 assays on two independent tetraploid cell lines. Figure 5: DNA methylation silencing of p21 uncouples p53 activation and p21 expression. ( a ) Western blot analyses of levels of the nuclear form of p53, phosphorylated p53 (P-p53), and p21 in the normal diploid and aneuploid cancer cells. ( b ) DNA methylation status in the promoter regions of p21 ( Cdkn1a ) in aneuploid cancer cells and normal diploid cells. DNA methylation status is indicated by the Log 2 value of the hybridisation signal from the enriched methylated genomic DNA (MIRA) normalised with that from the input genomic DNA (INPUT). Black bars, hybridisation signals; grey bar, location of CpG islands. The DNA methylation profiling data accession number: GSE18815. ( c , d ) Near-polyploid aneuploid cancer or diploid normal cells ( n =3 for each type) were treated with 5′ AzadC (500 ng ml −1 ) for 48 h. The mRNA ( c ) and protein levels ( d ) of p21 in the 5′ AzadC-treated or untreated cells were analysed by quantitative PCR and western blot analysis, respectively. ( e) Aneuploid cancer or diploid normal cells were treated with 5′ AzadC (0, 100, or 500 ng ml −1 ; 48 h). Live cells were counted, and the relative growth rate calculated by dividing the number of cells by the number of the untreated cells (mock). Values are means±s.d. of three independent assays. ( f ) Aneuploid cancer cells were pretreated with control or p21 siRNA then cultured in the absence or presence of 500 ng ml −1 5′ AzadC for 48 h. The cell number was counted and the relative growth rate was calculated by dividing the number of cells under varying treatments by the number of cells treated with control siRNA oligos only. ( g ) Near-polyploid aneuploid cancer cells expressing GFP or GFP-p21 were seeded in 96-well plates (4,000 each well). Cell growth was monitored by CellTiter 96 Aqueous One Solution Cell Proliferation Assay kit every 24 h for 72 h. The relative cell number was calculated by comparison of the absorbance value at 570 nm (A570) of each well. The relative cell number of the wells with the cells expressing GFP only at 24 h was set as 100. Values are mean±s.d. of n =5 assays on two independent tetraploid cell lines. Full size image Aneuploid cancer cells were also found to be resistant to exogenous cytotoxic insults, including tumour necrosis factor (TNF)α ( Fig. 6a ), which induces p53-depedent senescence and apoptosis [34] , [35] . However, addition of 5′ AzadC greatly sensitised the aneuploid cancer cells to TNFα-mediated cytotoxic effects ( Fig. 6b ). This finding provided additional evidence that the epigenetic silencing of p21 and other p53-mediated senescence or apoptosis genes is a critical mechanism that allows the aneuploid cancer cells to escape p53-mediated proliferation barriers. To investigate if this result was also true in vivo , 5′ AzadC was administered to NOD/SCID mice (500 ng g −1 body weight for 5 days) that were injected with WT/FFAA aneuploid cancer cells. Treatments with 5′ AzadC significantly decreased the size of aneuploid-associated tumours compared with untreated NOD/SCID controls ( Fig. 6c ). 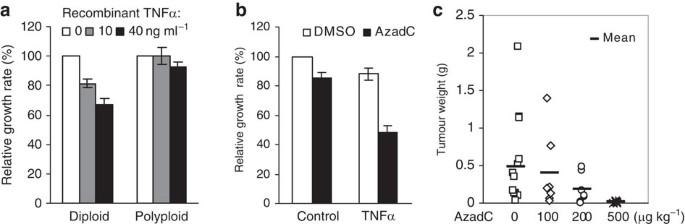Figure 6: The DNA methylation inhibitor 5′ AzadC restores p53-mediated growth arrest of near-polyploid aneuploid cancer cells. (a) Aneuploid cancer cells were resistant to TNFα-mediated growth arrest. Proliferation of aneuploid cancer or normal diploid cells in the presence of indicated concentrations of recombinant mouse TNFα was assessed. (b) Growth of aneuploid cancer cells treated with 40 ng ml−1TNFα in the absence or presence of 100 ng ml−15′ AzadC for 72 h. In panels (a) and (b), live cells were counted and the relative growth rate calculated by dividing the number of cells by the number of untreated cells (mock). Values are mean±s.d. of three independent assays. (c) 5′ AzadC inhibits aneuploid cancer growthin vivo. Tumour weights of NOD/SCID mice that first received 5×106aneuploid tumour cells (from clone C21), and were then treated with PBS buffer (control) or 5′ AzadC (100, 200 or 500 ng g−1body weight;n=15 for the control group,n=8 for each treatment group) for 5 consecutive days. Figure 6: The DNA methylation inhibitor 5′ AzadC restores p53-mediated growth arrest of near-polyploid aneuploid cancer cells. ( a ) Aneuploid cancer cells were resistant to TNFα-mediated growth arrest. Proliferation of aneuploid cancer or normal diploid cells in the presence of indicated concentrations of recombinant mouse TNFα was assessed. ( b ) Growth of aneuploid cancer cells treated with 40 ng ml −1 TNFα in the absence or presence of 100 ng ml −1 5′ AzadC for 72 h. In panels ( a ) and ( b ), live cells were counted and the relative growth rate calculated by dividing the number of cells by the number of untreated cells (mock). Values are mean±s.d. of three independent assays. ( c ) 5′ AzadC inhibits aneuploid cancer growth in vivo . Tumour weights of NOD/SCID mice that first received 5×10 6 aneuploid tumour cells (from clone C21), and were then treated with PBS buffer (control) or 5′ AzadC (100, 200 or 500 ng g −1 body weight; n =15 for the control group, n =8 for each treatment group) for 5 consecutive days. Full size image Polyploidisation promotes cancer progression in vivo We previously showed that the WT/FFAA mice developed high frequency of lung adenoma and adenocarcinoma [6] . It has been suggested that mutations in oncogenes including EGFR and Kras can initiate lung tumours [36] , [37] , [38] . Supporting this hypothesis, we found that of the ten WT/FFAA lung tumours we examined, two tumours carried the L705S or K738N mutations in the EGFR gene, and another two tumours had the G12D mutation in the Kras gene, which frequently occurs in human and mouse lung cancers [36] , [37] , [38] . However, hyper-DNA replication in the newly initiated tumour cells due to oncogene mutations can cause DNA replication stresses, especially if the cells already carry mutations in DNA replication genes, such as FEN1 . To investigate if the formation of polyploidy and subsequent aneuploidy contributed to overcoming such replication stresses in vivo , we first employed a dual-colour fluorescence in situ hybridisation (FISH) to detect aneuploid cells carrying three or more copies of both chromosome 2 and chromosome 8 in tissue sections of lung adenoma ( n =8) and adenocarcinoma ( n =10) from WT/FFAA mice. The adenocarcinoma but not adenoma had a significant amount of such aneuploid cells ( Fig. 7a and Supplementary Fig. S11a ). To further verify that polyploidisation was associated with tumour expansion and progression in vivo , we isolated single cells from a pool of small (1–2 mm) or large lung tumours (4–5 mm), which are predominantly lung adenoma or adenocarcinoma, respectively, according to previous histological analysis [6] , [38] . FACS-analysis revealed that the adenoma cells were diploid or near diploidy, whereas the adenocarcinoma cells were near-polyploid aneuploidy ( Fig. 7b and Supplementary Table S3 ). We noticed the G1/G0 peak of adenocarcinoma were relatively broader than that of the normal lung or adenoma, indicating that the population might contain heterogeneous aneuploid cells. In addition, aneuploid adenocarcinoma cells had a higher S/G2 cells than the diploid normal or adenoma cells ( Fig. 7b and Supplementary Table S3 ). Moreover, lung adenocarcinoma had significantly less TUNEL (terminal deoxynucleotidyl transferase dUTP nick end labelling)-positive cells than lung adenoma ( Fig. 7c,d and Supplementary Fig. S11b ). The lung adenocarcinoma also had less X-gal-positive cells, which is indicative of cellular senescence [39] , than the lung adenoma ( Fig. 7e,f and Supplementary Fig. S11c ). 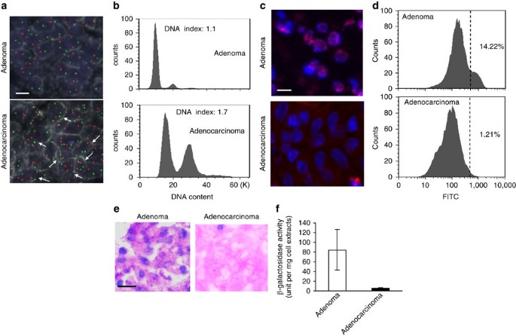Figure 7: Malignant adenocarcinoma in WT/FFAA mice was associated with near-polyploid aneuploidy and reduced apoptosis. (a)In vivolevels of aneuploidy of lung adenoma (n=8) and adenocarcinoma (n=10) were analysed with dual-colour interphase FISH (probes 2qA1 (red, chromosome 2) and 8qA1 (green, chromosome 8)). Aneuploid cells with three or more copies of chromosomes 2 and 8 are indicated by white arrows. Scale bar equals 20 μm. (b) FACS analysis of cells isolated from normal lung, adenoma (a pool of eight tumours of 1–2 mm diameters), and adenomcarcinoma (tumours of 3–5 mm diameters), following a previously published protocol51. The data was processed using the FlowJo software. DNA index was determined by comparing the position of the G1/G0 peak of adenoma or adenocarcinoma with that of the normal lung cells (diploid). (c) TUNEL staining (red) of apoptotic cells in tissue sections of the lung adenoma (n=8) or adenocarcinoma (n=10). Nuclei were stained with DAPI (blue). Pink spots were counted as TUNEL-positive nuclei. Scale bar equals 25 μm. (d) Tumour cells isolated from normal lung (negative control), adenoma (a poll of eight small tumours with diameters of 1-2 mm) or adenocarcinoma (a pool of three large tumours with diameters of 3–5 mm) were stained with APO-DIRECT kit (TUNEL assay). Cells with FITC intensities that were greater than 500 were considered as apoptotic cells (Supplementary Fig. S12). Dotted lines: Cutoff for quantification of apoptotic cells. (e) X-gal staining (blue) of senescent cells in the tissue sections of lung adenoma (n=8) or adenocarcinoma (n=6). The cytoplasm was counterstained with eosin solution (red). Tumours with at least ten blue spots, as shown for adenoma, were considered X-gal-positive. Scale bar equals 50 μm. (f) Mammalian β-galactosidase activity in the cell extracts from the lung adenoma or adenocarcinoma were assayed by the mammalian β-galactosidase activity assay kit (Thermo Scientific). One unit β-galactosidase activity was arbitrarily defined as an increase of 0.001 of absorbance 405 nm (A405) per hour. Values are mean±s.d of assays using three independent cell extracts. Figure 7: Malignant adenocarcinoma in WT/FFAA mice was associated with near-polyploid aneuploidy and reduced apoptosis. ( a ) In vivo levels of aneuploidy of lung adenoma ( n =8) and adenocarcinoma ( n =10) were analysed with dual-colour interphase FISH (probes 2qA1 (red, chromosome 2) and 8qA1 (green, chromosome 8)). Aneuploid cells with three or more copies of chromosomes 2 and 8 are indicated by white arrows. Scale bar equals 20 μm. ( b ) FACS analysis of cells isolated from normal lung, adenoma (a pool of eight tumours of 1–2 mm diameters), and adenomcarcinoma (tumours of 3–5 mm diameters), following a previously published protocol [51] . The data was processed using the FlowJo software. DNA index was determined by comparing the position of the G1/G0 peak of adenoma or adenocarcinoma with that of the normal lung cells (diploid). ( c ) TUNEL staining (red) of apoptotic cells in tissue sections of the lung adenoma ( n =8) or adenocarcinoma ( n =10). Nuclei were stained with DAPI (blue). Pink spots were counted as TUNEL-positive nuclei. Scale bar equals 25 μm. ( d ) Tumour cells isolated from normal lung (negative control), adenoma (a poll of eight small tumours with diameters of 1-2 mm) or adenocarcinoma (a pool of three large tumours with diameters of 3–5 mm) were stained with APO-DIRECT kit (TUNEL assay). Cells with FITC intensities that were greater than 500 were considered as apoptotic cells ( Supplementary Fig. S12 ). Dotted lines: Cutoff for quantification of apoptotic cells. ( e ) X-gal staining (blue) of senescent cells in the tissue sections of lung adenoma ( n =8) or adenocarcinoma ( n =6). The cytoplasm was counterstained with eosin solution (red). Tumours with at least ten blue spots, as shown for adenoma, were considered X-gal-positive. Scale bar equals 50 μm. ( f ) Mammalian β-galactosidase activity in the cell extracts from the lung adenoma or adenocarcinoma were assayed by the mammalian β-galactosidase activity assay kit (Thermo Scientific). One unit β-galactosidase activity was arbitrarily defined as an increase of 0.001 of absorbance 405 nm (A405) per hour. Values are mean±s.d of assays using three independent cell extracts. Full size image DNA SSBs arise and persist due to genetic defects in DNA replication and repair genes, including FEN1 . The FFAA FEN1 mutation disrupting the FEN1/PCNA interaction causes defects in DNA replication and repair, and results in DNA SSBs in the genome [6] . Consistently, mutations at the R192 residue, including R192Q, a FEN1 SNP present in the human genome ( http://www.ncbi.nlm.nih.gov/projects/SNP/ ), that also disrupt the FEN1/PCNA interaction, result in DNA strand breaks (Guo et al . [2] ). In addition, we have identified a group of FEN1 mutations, which eliminate the exonuclease activity of FEN1 and are present in human cancers [38] . More recently, we have shown that mouse cells carrying the E160D mutation that models this class of nuclease-deficient mutants, display BER defects and accumulate DNA SSBs in response to the DNA mutagen methylnitrosourea [40] . It is known that unrepaired SSBs may collapse DNA replication forks, resulting in DNA replication stresses and DSBs [1] , [5] , [40] . Meanwhile, oncogenesis also induces DNA replication stresses, which activate ATM/ATR and p53, and lead to cellular senescence. These molecular mechanisms have been thought to prevent early tumour progression [11] , [12] , [41] . Therefore, the initiated tumour cells must adapt to or reduce the DNA replication stresses to progress to malignancy. In support of this hypothesis, recent studies indicate that carcinoma has a considerably lower DNA damage response index than the corresponding precancerous lesion [11] , [42] , [43] . Our current studies consistently revealed that in unrestrictedly proliferating tumour cells, ATR-mediated DNA damage responses and cellular senescence were greatly reduced. In addition, WT/FFAA lung adenoma cells, but not adenocarcinoa, were associated with high levels of senescence and apoptosis. We further suggest the formation of tetraploidy and aneuploidy, which is a hallmark of human cancer [24] , [44] , [45] , is a key molecular mechanism that enables tumour cells to overcome DNA replication stresses and bypass the p53-mediated cell death pathways to acquire unlimited proliferation potential ( Fig. 8 ). In our current study, a very striking cellular phenotype observed in the in vitro expansion assays was that all unlimitedly proliferating WT/FFAA cells were near-polyploid aneuploid. In addition, lung adenoma from WT/FFAA mice was shown to be largely diploid, but lung adenocarcinoma was largely polyploid. These observations suggest that polyploidisation may positively affect cancer progression. Our single-cell gene expression profiling studies suggest that polyploidisation produces populations of cells with a wide spectrum of DNA damage response and repair gene networks. This would increase the chance that a subpopulation of the aneuploid tumour cells adapt or overcome replication stresses and bypass the p53-mediated cell death or senescence pathways, thereby evolving into malignant cancer cells. This hypothesis is consistent with the current view that cancer is a micro-evolutionary disease [46] . 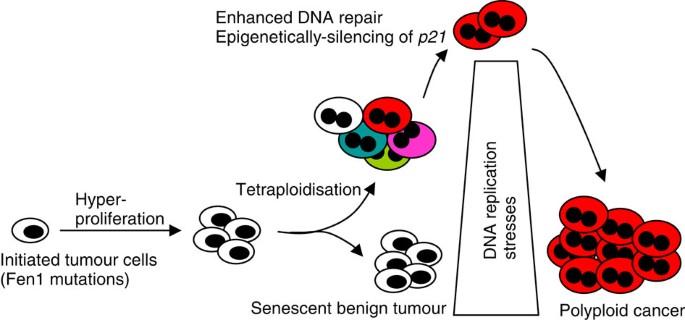Figure 8: A model of tetraploidy formation as a key molecular event for overcoming DNA replication stresses and malignant cancer progression. DNA replication stresses, which can occur due to mutations in DNA replication genes such as Fen1, environmental insults or oncogene activation, normally arrest the cell cycle and the senescence and apoptosis pathways serve as barriers to prevent tumour cell progression. At the same time, DNA replication and repair defects frequently result in the formation of tetraploidy and polyploidy. This leads to populations of genetically and epigenetically heterogeneous cells represented by different colours (white, red, pink, green, or blue). We observed subpopulations of polyploid cells with overexpression of BRCA1, p19arf and other DNA repair genes that reduce DNA replication stresses, and DNA methylation silencing of p53 downstream targets to escape senescence and apoptosis, and proposed these cells undergo clonal expansion (red cells). Figure 8: A model of tetraploidy formation as a key molecular event for overcoming DNA replication stresses and malignant cancer progression. DNA replication stresses, which can occur due to mutations in DNA replication genes such as Fen1, environmental insults or oncogene activation, normally arrest the cell cycle and the senescence and apoptosis pathways serve as barriers to prevent tumour cell progression. At the same time, DNA replication and repair defects frequently result in the formation of tetraploidy and polyploidy. This leads to populations of genetically and epigenetically heterogeneous cells represented by different colours (white, red, pink, green, or blue). We observed subpopulations of polyploid cells with overexpression of BRCA1, p19arf and other DNA repair genes that reduce DNA replication stresses, and DNA methylation silencing of p53 downstream targets to escape senescence and apoptosis, and proposed these cells undergo clonal expansion (red cells). Full size image We have shown that WT/FFAA aneuploid cancer cells with upregulated BRCA1- and p19arf-mediated DNA damage response and repair gene networks are selected for clonal expansion, suggesting an important role for these two proteins in coping with DNA replication stresses. BRCA1 interacts with Rad51 to promote DSB repair via the HR pathway [8] , [17] , [18] , [19] , [20] . In addition, BRCA1 has been shown to promote NHEJ activity [19] . The p19arf has been shown to stabilise p53, which mediates DNA repair, cellular senescence and apoptosis [21] , [47] . Here, our data suggest new, critical roles for BRCA1 and p19arf in SSB repair and the reduction of DNA replication stresses. Our in vitro assays using purified recombinant proteins demonstrated that p19arf strongly stimulated both Polδ- or Polβ-mediated gap filling and FEN1-mediated flap cleavage, and BRCA1 also enhanced flap cleavage by FEN1. Because gap filling and flap cleavage are important steps in both the DNA SSB repair and NHEJ repair pathways [1] , [5] , [26] , BRCA1 and p19arf may promote DNA SSB and NHEJ activity. A decrease in the DNA SSBs would reduce the frequency of collapsed DNA replication forks, thereby attenuating DNA replication stress response. The enhanced NHEJ activity should facilitate the repair of DSBs to suppress DNA damage response pathways that lead to cellular senescence. However, this may also increase improper repair of many one-ended DNA DSBs leading to chromosomal translocations and genome instabilities. Both BRCA1 and p19arf can activate p53, which induces the expression of p21 and other genes to arrest the cell cycle and trigger senescence or apoptosis [21] , [22] , [23] , [29] . Therefore, inactivation of these p53-mediated pathways may be critical for cells to progress towards malignancy. Mutations in p53 occur in approximately 50% of human cancers, and it is proposed to be a key mechanism enabling tumour cells to escape p53-mediated cellular senescence or apoptosis [29] , [48] , [49] . Here we suggest that DNA methylation at the promoter regions of p21 and other p53 target genes can also act to silence the p53 pathways, and results in a unique response to DNA replication stress, allowing the aneuploid cancer cells to promote DNA repair to prevent breakage-mediated cell death, but escaped cellular senescence and apoptosis ( Fig. 8 ). In addition, we suggest that DNA methylation-induced silencing of the p53 pathways allows the aneuploid cancer cells to become resistant to exogenous cytotoxic insults, such as TNFα, which is secreted by immune cells to induce senescence and apoptosis via the p53 pathways [50] . This would in turn, further promote the in vivo progression of cells towards malignancy. Taken together, the results from our current study indicate that aneuploid cancer cells overcome DNA replication stresses by increasing DNA repair activity and escape senescence and apoptosis via epigenetic reprogramming of the p53-mediated senescence and apoptosis pathways rather than through p53 mutation. Generation of limited and unlimited expansion transformed cells Spontaneously transformed cells were produced as previously described [6] . Briefly, 5×10 5 mouse primary MEFs (P1, E13.5) were seeded onto a 10-cm dish and cultured in Dulbecco's modified Eagle's medium supplemented with 10% fetal bovine serum for 15–25 days. Cells from each colony were picked, transferred and cultured in a 48-well plate. Once the culture reached 90% confluence, cell numbers were counted and all cells were transferred to a 24-well plate. Likewise, the cells were passed to a 12-well or 6-well plate, or a 10-cm dish. If cells from a clone continuously expanded with similar or higher proliferation rates after six additional passages in the 10-cm dish, we considered them to be an unlimited expansion clone. Those that did not continue to proliferate under these conditions were considered to be limited expansion clones. Tumour grafting in NOD/SCID mice Aneuploid cancer cells (5×10 7 ) were subcutaneously injected into NOD/SCID mice (2 months old, n =3 for each cell line). For the 5′ AzadC experiments, NOD/SCID mice that were injected with aneuploid cancer cells were also treated with 5′ AzadC daily for 5 days (0, 100, 200, 500 ng g −1 body weight, 100–200 μl injection volume). All mice were observed for 2 months. The mice were then killed, and subcutaneous tumours were dissected and weighed. All protocols involving animals were approved by the Research Animal Care Committee of City of Hope, in compliance with the Public Health Service Policy of the United States. Recombinant protein Recombinant human FEN1, Polδ and Polβ were expressed and purified as previously described [6] , [52] . Purified recombinant human BRCA1 was purchased from Active Motif. To express and purify human p14arf (the human homologue of mouse p19arf), a pcDNA-myc-ARF plasmid, which encodes a c-myc-tagged human p14arf [53] , was transfected into 293T cells. After 48 h additional culturing, the cells were harvested and lysed. The c-myc-tagged p14arf was purified by the affinity purification kit for the c-myc tagged protein, according to the manufacture's instruction (MBL International). The eluted c-myc-tagged p14arf was examined by SDS–PAGE and verified by western blotting analysis ( Supplementary Fig. S13 ), using an antibody against human p14arf (Santa Cruz Biotchnologies). In vitro DNA SSB repair and NHEJ assays SSB repair on the gapped DNA substrate with or without a DNA–RNA flap was assayed as previously described [6] , [54] . Briefly, NEs were prepared and mixed with DNA substrates (1 pmol) in reaction buffer A (50 mM Hepes-KOH, pH 7.5, 45 mM KCl, 5 mM MgCl 2 , 1 mM dithiothreitol, 0.1 mM EDTA, 2 mM ATP, 200 units creatine-phosphokinase, 0.5 mM NAD and 5 mM phosphocreatine). Each reaction (15 μl) also contained 5 μCi [α- 32 P] dCTP and 50 μM each of dATP, dGTP and dTTP. NHEJ was assayed as previously described [19] , [28] . A 3′ end- 32 P-labeled oligo-based DNA duplex was prepared. There was a two-nucleotide (–GG) overhang at the non-labeled 3′-end of the DNA substrate to resemble non-compatible DNA end joining [28] . NEs were incubated with DNA substrates (1 pmol) in the reaction buffer (50 mM triethanolamine–HCl, pH 7.5, 5 mM Mg(OAc)2, 80 mM potassium acetate, 2 mM ATP, 1 mM dithiothreitol and 100 μg ml −1 BSA) containing 50 μM each of the four deoxyribonucleotides. SSB repair or NHEJ reactions were carried out for the indicated times at 37 °C, and the product was analysed with 15 or 6% denaturing PAGE and autography. Metaphase spread preparation and analysis Cells treated with colcemid (0.1 μg ml −1 , 4 h) were harvested, washed with PBS buffer and incubated with hypotonic solution (75 mM KCl). Cells were then fixed with Carnoy's solution and dropped onto a glass slide, which was then baked (65 °C, overnight), stained with a Giemsa solution, scanned under a microscope (Olympus AX70) for mitotic cells and imaged using Image Pro 6.3 (Media Cybernetics, Inc.). The chromosome number of each mitotic cell was analysed and scored using Image Pro 6.3. Typically, 100–200 mitotic cells were analysed. Immunofluorescence staining To stain for phospho-Chk1, phospho-ATR or γH2AX, MEFs grown on glass cover slides were fixed with 4% paraformaldehyde, permeabilised with 0.1%. Triton X100, blocked with Image iT FX signal enhancer (Invitrogen) and incubated (1.5 h, room temperature) with the indicated primary antibodies. Antibodies against phospho-Chk1 (S345; 1:400) and γH2AX (1:400) were from Abcam, and the antibodies against phospho-ATR (1:200) and phospho-ATM (1:200) were from Cell Signaling Technology. Cells were then washed with PBS buffer and incubated (1 h, room temperature) with corresponding secondary antibodies (1:200, Invitrogen). Slides were washed with PBS buffer, counter stained with DAPI and analysed with a fluorescence microscope (Olympus AX70). Detection of senescent cells Senescent cells were detected by staining for X-gal-positive cells as previously described [39] . The X-gal staining kit was from Cell Signaling. Briefly, cells cultured in 12- or 6-well plates were fixed (10% formalin in PBS) for 10 min. After being washed with PBS buffer, fixed cells were incubated (overnight, 37 °C) with the X-gal staining solution. Cells were then analysed with an inverted light microscope (IX81, Olympus). mRNA microarray analysis For microarray analysis, total RNA was extracted from parental MEFs (WT/FFAA, P1, E13.5, diploid normal control) and cells from clones with limited or unlimited expansion ( n =3 independent lines for each group) using the Qiagen RNaeasy kit (Qiagen). The Affymetrix GeneChip Mouse Gene 1.0-ST array (Affymetrix, Santa Clara, CA) was used to define gene expression profiles from the samples. Biotinylated single-stranded cDNA was generated using 100 ng total RNA according to the manufacturer's protocol. Hybridisation cocktails containing 2.5 μg fragmented, end-labeled cDNA were prepared and applied to the GeneChip and incubated for 16 h. Arrays were washed and stained with the GeneChip Fluidics Station 450 using FS450_0007 script. They were then scanned at 5-μm resolution using the Affymetrix GCS 3000 7G and GeneChip Operating Software v. 1.4 to produce CEL intensity files. Raw intensity measurements of all probe sets were background-corrected, normalised and converted into expression measurements using Affymetrix's Expression Console v1.1.1. The Bioconductor 'LIMMA' package was then used to identify genes differentially expressed between the tetraploid and diploid samples. Significant genes were selected using a cut-off of P <0.05 and fold change of 2. Data were analysed with DAVID (Database for Annotation, Visualization and Integrated Discovery) functional annotation tools and Ingenuity Pathway analysis program to identify statistically significant diseases, gene networks and pathways that were upregulated or downregulated in transformed cells with limited or unlimited expansion potential and compared witho the diploid control. DNA methylation analysis DNA methylation in aneuploid cancer cells and normal diploid cells was analysed with MIRA [55] . Briefly, sonicated genomic DNA (approximately 500 bp) was incubated with the methylated DNA-binding proteins MBD2B and MBD3L1 to pull down methylated DNA. Enriched methylated and input genomic DNA samples were quantitatively amplified by real-time PCR and labeled with Cy3 and Cy5, respectively. The labeled DNA fragments were hybridised to the Nimblegen HG18 CpG Promoter array (Roche Nimblegen). Normalised hybridisation signals were analysed with SignalMap (Nimblegen). Methylated CpG islands shown in SignalMap were then verified by Bisulfite DNA sequencing [55] . DNA methylation inhibitor treatment WT/FFAA aneuploid cancer cells or normal diploid cells were treated as indicated with the DNA methylation inhibitor, 5-aza-2′-deoxycytidine (5 'AzadC) [56] . Expression of p21 and CXCL2 was determined by quantitative real-time PCR (Taqman gene expression assays, Applied Biosystems) and western blot. The corresponding cell growth rate was measured by cell counting. Histopathology and staining To conduct histopathology analysis, fixed (10% formalin) or frozen tissue sections were stained with haematoxylin and eosin. To determine the ploidy status of cells in tumour tissues, dual-colour FISH for chromosomes 2 and 8 was conducted with FISH probes that corresponded to the mouse chromosomes 2qA1 and 8qA1. Slides were analysed with a BioView Imaging system (BioView, UK). To stain DNA strand breaks, paraffin-embedded tissue sections (5 μm) were de-waxed with xylene (5 min) and rehydrated in an ice-cold ethanol series (100, 95, 75 and 50%; 2 min each). Sections were permeabilised with 0.1 M sodium citrate and 0.1% Triton X-100 (8 min). Slides were then incubated (1 h, 37 °C) with TUNEL staining solution (Roche), washed with PBS and examined with a fluorescence microscope (Olympus AX70). To stain senescent cells in lung tumour tissue, frozen tissue sections (5 μm) were fixed with 1% formalin and stained with X-gal staining solution (Cell Signaling) at 37 °C overnight. Cytoplasm was stained with eosin Y solution (Sigma). All slides for each staining were analysed in a double-blind fashion. Accession codes: The microarray data have been deposited in the GEO database under accession code GSE18815 . How to cite this article: Zheng L. et al . Polyploid cells rewire DNA damage response networks to overcome replication stress-induced barriers for tumour progression. Nat. Commun. 3:815 doi: 10.1038/ncomms1825 (2012).